Sample sequencing of vascular plants demonstrates widespread conservation and divergence of microRNAs Small RNAs are pivotal regulators of gene expression that guide transcriptional and post-transcriptional silencing mechanisms in eukaryotes, including plants. Here we report a comprehensive atlas of sRNA and miRNA from 3 species of algae and 31 representative species across vascular plants, including non-model plants. We sequence and quantify sRNAs from 99 different tissues or treatments across species, resulting in a data set of over 132 million distinct sequences. Using miRBase mature sequences as a reference, we identify the miRNA sequences present in these libraries. We apply diverse profiling methods to examine critical sRNA and miRNA features, such as size distribution, tissue-specific regulation and sequence conservation between species, as well as to predict putative new miRNA sequences. We also develop database resources, computational analysis tools and a dedicated website, http://smallrna.udel.edu/ . This study provides new insights on plant sRNAs and miRNAs, and a foundation for future studies. MicroRNAs (miRNAs) are a class of 20–24 nucleotide small RNA (sRNA) sequences that regulate gene expression in eukaryotes, from single cell green algae to mammals [1] , [2] , [3] . MiRNAs are transcribed from genomic loci as messenger RNA precursors, which fold into a stem-loop secondary structure that undergoes cleavage by endonucleases (Drosha RNAse III in animals, DICER-like in plants), resulting in the production of the mature miRNA sequence [2] , [4] . MiRNAs are classified into families according to the nucleotide sequence of the mature form, with identical or very similar sequences grouped into the same family. Studies of plant miRNAs have historically focused on sequence conservation and, more recently, miRNA loci sequence variability across species [5] , [6] . Several of these studies have shown that only a small number of miRNA families are present across phylogenetically distant species [3] , [5] . These conserved miRNAs predate the divergence of gymnosperms and angiosperms 305 million years ago, and the divergence between vascular plants and mosses 490 million years ago [7] . Functionally, plant miRNAs are involved in many fundamental biological processes, and their conservation across the plant kingdom suggests that these molecules have been active in the regulation of gene expression and have played key roles in plant developmental processes since the earliest stages of their evolution [8] , [9] . Nevertheless, the majority of miRNA sequences are only present in one to a few species [3] , [10] , [11] , [12] , and a comparison between Arabidopsis thaliana and A. lyrata shows that even closely related species do not have highly overlapping miRNomes [6] . This suggests that many miRNA loci have emerged recently, and that miRNA loci in plant genomes are in a constant dynamic evolutionary state [6] , [11] , [12] . With the advent of next-generation sequencing technologies, an impressive amount of sRNA sequencing data is now available in public databases. However, despite the extensive available resources on plant sRNAs, a comprehensive comparative analysis of miRNA sequences across the plant kingdom has not been performed. In this work we examined sRNA data from 34 plant species, ranging from green algae to eudicots. Analysis of these sequence data, and the abundances of the sequences contained therein, revealed new information on miRNA conservation, divergence and sequence variability, and the correlation of such characteristics with sequence abundance. We observed that very few miRNA sequences, all of high abundance, are conserved across most analysed species, while the majority of miRNAs are species specific, of low abundance, and correspond to substitution variants of the reference plant miRBase sequences. We further show that a sequence abundance comparison across species is a simple yet powerful methodology that can reveal miRNA substitution variants as putative new miRNA sequences, all without the need for a genomic reference. Selection and sequencing of plant specimens To understand miRNA sequence diversity in the plant kingdom, we developed and analysed a set of sRNA libraries from 34 plant species, from green algae to non-seed to seed plants. For each species, up to three samples from different organs, tissues, developmental stages or treatments were analysed, resulting in 99 sRNA sequencing libraries. The species panel included most plants for which extensive genomic resources are currently being developed, and was complemented by a panel of diverse species that represent important families or nodes of the plant kingdom. The 34 species were represented by 3 green algae, 1 fern, 3 orders of gymnosperms, 3 basal angiosperms, 9 monocots and 14 eudicots ( Fig. 1 ; Supplementary Data 1 ). Among the selected species are economically important crops, and representatives of grasses and tree species that are valuable sources of wood and/or biofuel products. Two major plant families, Poaceae and Solanaceae, included a large set of species and were emphasized because their genomic sequences have been a high priority for the plant genomics community. In addition, these plants are among the most important botanical species for their extensive use by humans. Finally, two species of increasing scientific importance, Mimulus guttatus (monkey flower) and Silene latifolia (white campion), were further included as model organisms for ecological genomics and sex-chromosome evolution, respectively [13] , [14] . Thus, the selected species were broadly representative of the diversity of the Viridiplantae (green plants). 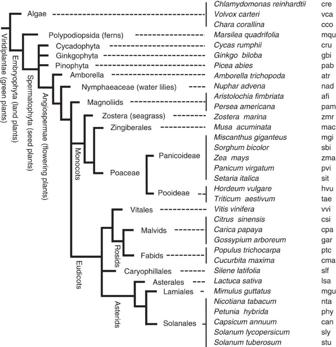Figure 1: Phylogenetic distribution of the 34 plant species analysed in this study. Phylogeny was adapted from the Tree of Life Web Project (http://www.tolweb.org/tree/). In all subsequent figures, species are presented in the order shown here, using the three-letter codes to the right of the full species name. Figure 1: Phylogenetic distribution of the 34 plant species analysed in this study. Phylogeny was adapted from the Tree of Life Web Project ( http://www.tolweb.org/tree/ ). In all subsequent figures, species are presented in the order shown here, using the three-letter codes to the right of the full species name. Full size image With few exceptions, we examined both leaves and the reproductive organs (for example, flowers in Angiosperms) from all of the higher plants investigated ( Supplementary Data 1 ). In addition, a third sample was analysed for most species, and included either additional organs (for example, roots, pods), tissues from plants under biotic or abiotic stress or tissues of particular agronomic interest (for example, cotton fibres or poplar xylem). For green algae species, samples were obtained from three different growth conditions. As such, we expect this set of samples to contain the majority of miRNAs encoded in the genome of the corresponding species. sRNA sizes across the plant kingdom Sequencing of the sRNAs obtained from the above-mentioned materials resulted in a median of 3.9 million reads, and 1.2 million distinct sequences per library. All libraries combined represented 461 million sRNAs, with 132 million unique sRNA sequences in total. We first examined the size distribution of the sRNAs present in our sequencing libraries. Plant sRNAs are typically found in two predominant size classes, 21 nucleotides and 24 nucleotides. The former was classically considered to comprise miRNAs and trans -acting short interfering RNAs (tasiRNAs), and the latter heterochromatic siRNAs [15] . Recently, it has become clear that phased siRNAs can contribute to one or both of these major size categories depending on the plant [16] , [17] , [18] . While this pattern was observed consistently in angiosperms, non-angiosperm species included different patterns, such as a single, predominant 20–21 nucleotide size class for Chlamydomonas reinhardtii , a 21–22 nucleotide size class for Volvox carteri , a predominant 22 and 23 nucleotide size class for Chara corallina or a single predominant 21 nucleotide size class for non-angiosperm vascular plants ( Fig. 2 and Supplementary Fig. 1 ). Picea abies (Norway spruce) lacks 24 nucleotide sRNAs, and it has previously been reported that Pinus contorta also lacks 24 nucleotide siRNAs [19] , which suggests that this is a conserved feature of the Pinaceae family. However, the presence of a strong 24 nucleotide size class in Cycas rumphii , and a small, but still present 24 nucleotide size class in both Ginkgo biloba and in the fern Marsilea quadrifolia suggests that the 24 nucleotide class of sRNAs originated before gymnosperm diversification. 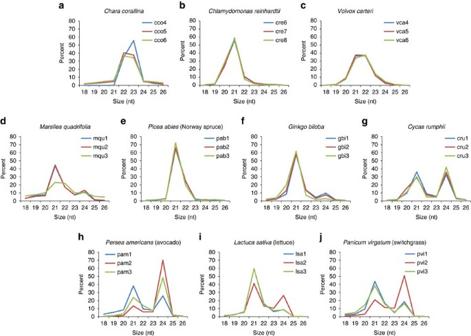Figure 2: Size distribution of sRNA sequences. Relative proportions of sRNA sequences are displayed as percentages for each size category in a representative subset of the analysed species. (a–c) Green algae; (d) ferns; (e–g) gymnosperms; (h–j) angiosperms. cco4: thallus in control conditions, cco5: nutrient starvation, cco6: nutrient starvation plus salt stress, cre6: control, cre7: phosphate starvation, cre8: sulphate starvation, vca4: control, vca5: sulphate starvation, vca6: phosphate starvation, mqu1: leaves, mqu2: roots, mqu3: drought-stressed leaves, pab1: needles, pab2: female cone, pab3: lateral bud meristem, gbi1: leaves, gbi2: female cone, gbi3: male cone, cru1: leaves, cru2: female cone, cru3: male cone, pam1: leaves, pam2: flowers, pam3: fruits, lsa1: leaves, lsa2: flowers, lsa3: leaves inoculated withBremia lactucae, pvi1: leaves, pvi2: flower, pvi3: drought-stressed leaves. Figure 2: Size distribution of sRNA sequences. Relative proportions of sRNA sequences are displayed as percentages for each size category in a representative subset of the analysed species. ( a – c ) Green algae; ( d ) ferns; ( e – g ) gymnosperms; ( h – j ) angiosperms. cco4: thallus in control conditions, cco5: nutrient starvation, cco6: nutrient starvation plus salt stress, cre6: control, cre7: phosphate starvation, cre8: sulphate starvation, vca4: control, vca5: sulphate starvation, vca6: phosphate starvation, mqu1: leaves, mqu2: roots, mqu3: drought-stressed leaves, pab1: needles, pab2: female cone, pab3: lateral bud meristem, gbi1: leaves, gbi2: female cone, gbi3: male cone, cru1: leaves, cru2: female cone, cru3: male cone, pam1: leaves, pam2: flowers, pam3: fruits, lsa1: leaves, lsa2: flowers, lsa3: leaves inoculated with Bremia lactucae , pvi1: leaves, pvi2: flower, pvi3: drought-stressed leaves. Full size image miRNA conservation across the plant kingdom We then aimed to investigate the abundance and conservation across species of our identified miRNA sequences. These identified miRNA sequences included sequences matching both reference miRNA and miRNA* sequences, and nucleotide substitution variants (also known as isomiRs). We first used our list of identified miRNAs ( Supplementary Data 2 ) to calculate the miRNA abundances in each sequencing library, which ranged from 1,411 reads per million (RPM) library reads (0.14% of all sRNAs) in the C. corallina control library to 408,730 RPM library reads (40.87%) in the M. guttatus leaf library ( Supplementary Fig. 2 ). We then calculated the number of distinct miRNA sequences present in each of the 34 plant species. The resulting data set ( Supplementary Data 3 ) contains 100,014 unique sequences, while the 67 Viridiplantae species represented in version 19 of miRBase [20] account for 3,228 unique mature sequences. Of the 100,014 unique sequences, only 897 (0.90%) were identical, 902 (0.90%) were shorter, 5,129 (5.13%) had extra bases and 2,361 (2.36%) were shifted relative to the matching miRBase mature plant sequence. The remaining 90,725 sequences (90.71%) were nucleotide substitution variants. Although sequences identified without mismatches (that is, non-nucleotide substitution variants) do not represent the majority of sequences, they do represent the majority of reads for almost all species ( Supplementary Fig. 3 ). An overview of sequence abundances in Supplementary Data 3 indicated that a major divide in miRNA evolution exists between algae and terrestrial plants. No higher-plant miRNAs were observed in C. corallina , a species that has been described as the green algae most closely related to land plants [21] , [22] . Although some sequences present in terrestrial species could be detected at low abundances in C. corallina , they either matched our r/t/sn/small nucleolar RNA (snoRNA) database (miR894 and miR6300 sequences), suggesting that they are not true miRNA sequences, or their abundance was always very low, usually less than 1 RPM, which suggested cross-contamination during sequencing, rather than the actual presence of such sequences. C. corallina samples were obtained at the gametophytic stage, and this could introduce a bias versus the mostly sporophytic samples from terrestrial plants. Still, no miRNA families common to both algae and terrestrial plants could be found in our data set. In addition, previous reports indicate that no miR156 or miR166 sequences could be detected in gel blots of C. corallina total RNA [23] , and the putative Chara miR165/miR166 target sequence contains five mismatches relative to the canonical miR166 sequence 5′-CCCCUUACUUCGGACCAGGCU-3′ (ref. 24 ). All these data suggest that the early evolution of complex multicellular body plans occurred independently of conserved higher plant miRNAs. We next explored miRNA conservation across terrestrial species. As contaminant sequences, either of algal or animal/virus origin (Methods) could be found at abundances in the single digits, miRNA families were qualified as present when their abundance was >10 RPM in at least one sequencing library. A total of 82 known miRNA families were found to be present across several terrestrial plants ( Fig. 3 ). These families were grouped depending on their distribution across lineages and species. Group 1 was ubiquitous and generally highly expressed across all terrestrial species. Group 2 families, although represented in all taxonomic lineages, were absent or present at very low abundance levels (less than 10 RPM) in some species. Beyond conserved families, the remaining groups were distributed across species with diverse lineage enrichment, such as families in group 8, which are predominant in Solanaceae species. In addition, variation in abundance levels was observed for some families within plant lineages, for example, miR162 in Poaceae or miR6149 in Solanaceae. The fern M. quadrifolia , the most basal vascular plant that we examined, was missing most miRNA families from groups 3 to 8, which are present in gymnosperm or angiosperm species. Grasses also have undergone loss or radically decreased expression of families present in group 3, and lack families from groups 4, 6 and most families of group 8, which appear to be lineage specific (eudicots for group 4, basal angiosperms for group 6 and Solanaceae for group 8).Curiously, we also observed recurrently the (near) absence of several miRNA families in the sea grass Zostera marina , for example, miR394 (group 2), miR827 (group 5) or miR444 (group 7), relative to all the other monocots analysed. This phenomenon is particularly intriguing regarding the early phylogenetic and physical separation of this sea grass from land monocots. Finally, group 6 families are particularly abundant in gymnosperm species, and differentiate this lineage from the other vascular plants. An overview of the presence of miRNA families across the phylogeny of terrestrial species is presented in Fig. 4 . Notably, miRNA families previously reportedly derived from common ancestor genes show different patterns of expression across the species panel, reflecting episodes of gene duplication followed by lineage-specific functional diversification (for example, miR159/miR319 (ref. 25 )) or complete loss in some taxonomic groups, as in the example of miR529 versus miR156 (ref. 3 ). In our data set, the miRNA superfamily including miR390, miR1432 and several other miRNAs related in sequence ( Fig. 3 ) exhibits the most diversified pattern of taxonomic distribution suggesting a complex evolutionary history. 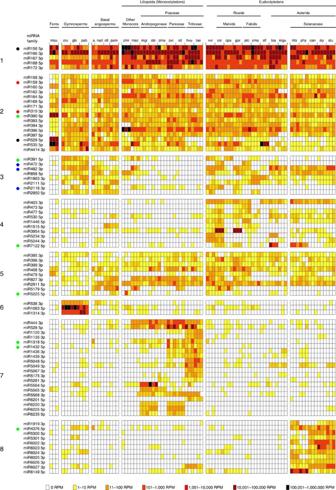Figure 3: Sequence abundance and conservation across Tracheophyta species. Abundance of 82 conserved miRNAs across the comparative panel of plant species and organs included in this study. Heatmap colours represent absolute normalized levels of miRNA expression ranging from 0 RPM (white) to 1,000,000 RPM (dark red) as indicated in the colour keys. MiRNA families are sorted in eight groups according to the degree of conservation and enrichment in the taxonomic groups analysed. 1, ubiquitous; 2, present in most taxonomic groups; 3, poorly enriched in monocots; 4, enriched in dicots; 5, enriched in angiosperms; 6, enriched in gymnosperms; 7, enriched in monocots; 8, enriched in Solanaceae. Coloured dots indicate related miRNA families. Figure 3: Sequence abundance and conservation across Tracheophyta species. Abundance of 82 conserved miRNAs across the comparative panel of plant species and organs included in this study. Heatmap colours represent absolute normalized levels of miRNA expression ranging from 0 RPM (white) to 1,000,000 RPM (dark red) as indicated in the colour keys. MiRNA families are sorted in eight groups according to the degree of conservation and enrichment in the taxonomic groups analysed. 1, ubiquitous; 2, present in most taxonomic groups; 3, poorly enriched in monocots; 4, enriched in dicots; 5, enriched in angiosperms; 6, enriched in gymnosperms; 7, enriched in monocots; 8, enriched in Solanaceae. Coloured dots indicate related miRNA families. 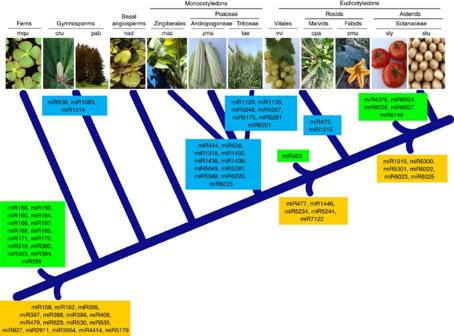Figure 4: miRNA family emergence across the phylogeny of terrestrial plant species. Families coloured green are conserved across virtually all corresponding species. Families coloured orange are conserved, although missing in a few corresponding species. Families coloured blue appear to be specific to a particular group of species. Full size image Figure 4: miRNA family emergence across the phylogeny of terrestrial plant species. Families coloured green are conserved across virtually all corresponding species. Families coloured orange are conserved, although missing in a few corresponding species. Families coloured blue appear to be specific to a particular group of species. Full size image Conservation of tasiRNA triggers We next used the sequences belonging to the 82 miRNA families presented in Fig. 3 to investigate the conservation of miRNA structural features, as size and 5′-nucleotide preference, both between miRNA families and between species. A miRNA size enrichment analysis was performed by clustering the 82 miRNA families in groups that emphasize different patterns of size distribution, based on the average expression level across all libraries ( Fig. 5 ). 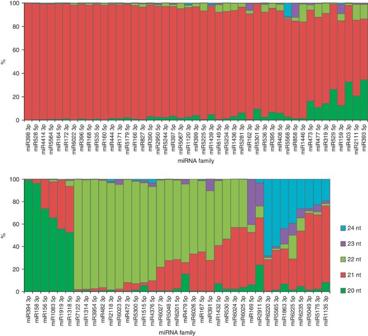Figure 5: Size distribution of conserved miRNA families. The relative abundance of different size categories, from 20 to 24 nucleotides, is shown for the 82 conserved miRNAs presented inFig. 3. Relative size contributions are reported for each miRNA family as an average of percent expression levels of each size across the panel of land plants analysed in this study. Figure 5: Size distribution of conserved miRNA families. The relative abundance of different size categories, from 20 to 24 nucleotides, is shown for the 82 conserved miRNAs presented in Fig. 3 . Relative size contributions are reported for each miRNA family as an average of percent expression levels of each size across the panel of land plants analysed in this study. Full size image Among the 82 conserved miRNA families presented in Fig. 3 , we were able to identify several miRNA families that have been reported to trigger the production of tasiRNAs. TasiRNAs are a class of secondary 21-nucleotide siRNAs that elicit sequence-specific cleavage of target transcripts similar to miRNAs but, in contrast with the latter, originate from the processing of tasiRNA transcripts after an initial cleavage by an independent miRNA. The ability of a miRNA to initiate the production of secondary siRNAs may be associated with structural asymmetry in the miRNA/miRNA* duplex, a condition that in most known cases is fulfilled when either a miRNA or a miRNA* is 22 nucleotide in size [26] , [27] . Twenty-one conserved miRNA families showed a prominent 22-nucleotide component ( Fig. 5 ), eight of these corresponding to known tasiRNA triggers, including miR167 (ref. 27 ), the miR472/482/2118 superfamily [16] , [28] , and the miR7122 and the related miR4376/1432/391 superfamilies [29] . Interestingly, a prevalence of 22-nucleotide species was also observed for miR479, whose sequence overlaps with the reverse complement of another tasiRNA initiator, miR171 (ref. 30 ), suggesting that it might represent the miRNA*. Additional miRNAs with a preference for a 22-nucleotide size were identified and sorted with those described above into different groups of taxonomic conservation ( Supplementary Fig. 4 ), although most of these have not been yet reported to initiate a cascade of secondary siRNAs. Among these we found miR1314, a family specific to gymnosperms (group 4), and several miRNAs that in our data set appear specific to either monocots (group 2) or Solanaceae (group 3). The remainder (group 1) show sparse distribution across species or erratic presence in a few of them, with miR167 as the only miRNA present in a 22-nucleotide form (but not exclusively) at a substantial expression level in nearly all samples. Other 22-nucleotide tasiRNA triggers are present in our data set but not at a high proportion in this size (miR168, miR393, miR396) or are not conserved at all (miR173, miR773). Among the tasiRNAs initiators targeting the TAS1 / 2 / 3 / 4 genes identified in A. thaliana (miR173, miR390 and miR828), miR390 is the only one present in all species and at high abundances in our data set. This miRNA is not expressed as a 22-mer but is thought to exert a trigger activity via its association with AGO7 (ref. 30 ). Interestingly, from an evolutionary perspective, miR390 is both highly conserved among higher plants and consistent in its size (21 nucleotides instead of the more canonical 22 nucleotides), representing a well-established, albeit minor, mechanism of tasiRNA initiation. Size distribution and starting nucleotide of miRNA families In 45 miRNA families, 21-mers were the most significant size class, accompanied in some cases by additional sizes, especially 20 nucleotide sequences ( Fig. 5 ). Six families exhibited a stronger preference for 20-mers, while in 21 families 22-mers were either the most abundant sequences or present in significant proportions. Ten families stood out for the presence of 23- or 24-mers at different degrees amid other sizes; six of the latter, miR1135, miR6220, miR6225, miR6235, miR5049 and miR5175, were monocot specific and such a limited conservation was expected in general for miRNA families with a broad size distribution typical of relatively young miRNAs [1] . Considering the predominance of 21-nucleotide long miRNAs, the persistence of a different size (for example, 20 or 22 nucleotide) in many taxonomic lineages may be suggestive of selective constrains. For example, while families like miR156 and miR168 show the coexistence of 20- and 21-nucleotide variants across the entire panel of samples investigated, we observed a predominant 20-nucleotide size for miR158 in nearly all samples where it is expressed ( Supplementary Fig. 5 ). It is unclear whether this size specificity has a functional consequence, like the 22-nucleotide preference of miR472/482/2118 associated with the generation of tasiRNAs. In other cases, size preference could have resulted from episodes of miRNA gene birth-and-death in critical points of plant evolutionary history. For instance, 22-mers of miR393 were negligible in all monocot samples, while miR167 22-nucleotide variants showed very low abundances, if any, in many dicots, although they were more abundant in all the other taxonomic groups ( Supplementary Fig. 5 ). Nucleotide composition at starting position is another critical feature of sRNAs correlated to their biogenesis and function [1] . In 61 of the 82 conserved miRNA families, the majority of sequences have a uracil at position 1, although some of these showed additional 5′-nucleotide composition to a variable degree. For the remaining 21 families, adenine, cytosine and even guanine were found in significant proportions at the 5′-position ( Fig. 6 ). 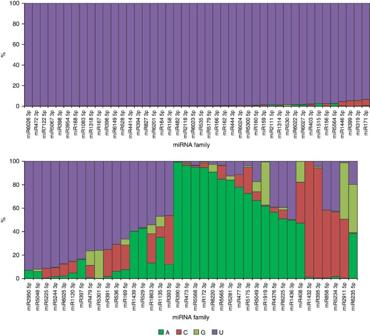Figure 6: 5′-nucleotide distribution of conserved miRNA families. Stacked bars represent the relative abundance of the 5′-nucleotide of all sequences for each of the 82 conserved miRNA families presented inFig. 3. Relative 5′-nucleotide usage is as an average of percent expression levels of each nucleotide across the panel of land plants analysed in this study. Figure 6: 5′-nucleotide distribution of conserved miRNA families. Stacked bars represent the relative abundance of the 5′-nucleotide of all sequences for each of the 82 conserved miRNA families presented in Fig. 3 . Relative 5′-nucleotide usage is as an average of percent expression levels of each nucleotide across the panel of land plants analysed in this study. Full size image A quick overview of miRBase sequences shows that many miRNAs belonging to the same family vary in the starting position of the mature miRNA. To assess the relative starting positions of our identified miRNAs in detail, we aligned the variants of each family and determined their most abundant starting positions across all libraries, with miRNA sequences further divided into size categories ( Supplementary Fig. 6 ). Out of the 45 miRNA families with a prevalence of 21-mers, 29 showed absolute or near-absolute preference for a single start position. In the remaining 16 families, secondary positions were relatively prominent, ranging in some cases between 20 and 67% of the frequency of the most represented start coordinate (for example, miR1446 or miR5281). In miRNA families where the contribution of multiple-size variants was considerable, size categories generally had overlapping starting positions (for example, miR530). The observation of a shift in the starting position among sequence variants of the same family suggested that the theoretical preconditions for functional diversification of miRNA families occurred to some extent during evolution. Therefore, we set out to investigate whether this phenomenon could be described as a random positional drift occurring at random in some species, or whether positional variants were distributed according to a taxonomic pattern. When the preferential starting positions of each miRNA were examined in each library, some miRNA families showed a pattern of positional differentiation between dicots and monocots, in particular miR396 and miR397 ( Supplementary Fig. 7 ). Indeed, miR396 variants starting at position 5 of the consensus are poorly represented in dicots compared with position 4 variants, but generally more abundant in monocot libraries, with a notable exception in Z. marina . The most frequent miR396 variant starting at position 5 is characterized by an insertion at position 6 of the mature miRNA, suggesting it is encoded by a distinct gene rather than being a shifted product processed from the same precursor. We also found preferential expression of two miR397 variants in monocots ( Supplementary Fig. 7 ), which start three nucleotides downstream relative to the non-monocot variant. Notably, both miR397 monocot variants are absent from the version 19 release of miRBase. As with the case of miR396, differences in start position highlight a new element of miRNA differentiation between lineages. In addition, the sequences at the two positions are overlapping and compatible with the generation of both variants from the same precursor(s) in two of the three grass species where genomic sequence was available for this analysis (rice, Brachypodium and sorghum). In other circumstances, taxonomic differentiation is the outcome of a more complex combination of factors. This is the case of miR393 where positional shift, size variation and 5′-nucleotide variation concur to diversify this miRNA family within grass species as well as between grasses and non-grass monocots ( Supplementary Fig. 7 ). Thus, miR393, together with miR396 and miR397, represent excellent examples for the investigation of sequence and structural determinants affecting the 5′-terminus of mature miRNA processed from the precursors. MiRNA sequence abundance and conservation are correlated We observed that all sequences belonging to 21 highly conserved families (groups 1 and 2 in Fig. 3 ) represent 54–98% of all miRNA sequences in almost all species ( Fig. 7a ). This suggested that abundant sequences correspond to sequences that are present in all terrestrial species. Indeed, miRNA abundance increases as the conservation of the sequence increases, with sequences detected in all 34 species we analysed having a median abundance three orders of magnitude higher than sequences present in a few species ( Fig. 7b ). 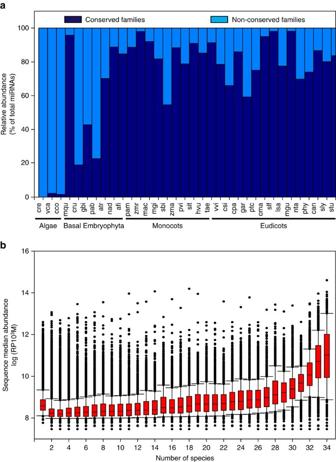Figure 7: Sequence conservation and abundance are correlated. (a) Conserved families make the majority of miRNAs. Stacked bars represent the sum of abundances of conserved (dark blue) and non-conserved (light blue) families across all analysed species. Abundances are expressed as the percentage of total miRNA abundances for each species. (b) Sequence abundance increases as its conservation across plant species increases. Each data point represents the abundance of a miRNA sequence present in the corresponding number of species. Box plots indicate the median (line), 25th and 75th percentiles (boxes), and 10th and 90th percentiles (whiskers) of sequence abundances. Dots represent outliers. Abundance is expressed as the base 10 logarithm of RP103M. The number of sequences per number of species was the following: 1: 60,733; 2: 38,385; 3: 19,453; 4: 13,653; 5: 10,701; 6: 8,917; 7: 7,533; 8: 6,897; 9: 5,824; 10: 4,901; 11: 4,401; 12: 4,057; 13: 3,992; 14: 3,781; 15: 3,841; 16: 3,425; 17: 3,180; 18: 3,241; 19: 2,680; 20: 2,801; 21: 2,458; 22: 2,135; 23: 2,646; 24: 2,401; 25: 2,476; 26: 2,445; 27: 1,783; 28: 2,017; 29: 1,944; 30: 1,771; 31: 3,256; 32: 993; 33: 793; 34: 443. Figure 7: Sequence conservation and abundance are correlated. ( a ) Conserved families make the majority of miRNAs. Stacked bars represent the sum of abundances of conserved (dark blue) and non-conserved (light blue) families across all analysed species. Abundances are expressed as the percentage of total miRNA abundances for each species. ( b ) Sequence abundance increases as its conservation across plant species increases. Each data point represents the abundance of a miRNA sequence present in the corresponding number of species. Box plots indicate the median (line), 25th and 75th percentiles (boxes), and 10th and 90th percentiles (whiskers) of sequence abundances. Dots represent outliers. Abundance is expressed as the base 10 logarithm of RP10 3 M. The number of sequences per number of species was the following: 1: 60,733; 2: 38,385; 3: 19,453; 4: 13,653; 5: 10,701; 6: 8,917; 7: 7,533; 8: 6,897; 9: 5,824; 10: 4,901; 11: 4,401; 12: 4,057; 13: 3,992; 14: 3,781; 15: 3,841; 16: 3,425; 17: 3,180; 18: 3,241; 19: 2,680; 20: 2,801; 21: 2,458; 22: 2,135; 23: 2,646; 24: 2,401; 25: 2,476; 26: 2,445; 27: 1,783; 28: 2,017; 29: 1,944; 30: 1,771; 31: 3,256; 32: 993; 33: 793; 34: 443. Full size image All species have thousands of unique miRNA sequences (except V. carteri , with 986 distinct sequences), with sequences with an abundance of less than 10 RPM representing 92 to 99% of the total. Only a few sequences per species had abundances over 10,000 RPM, and only four species had one sequence each with an abundance of 100,000 RPM or higher ( Fig. 8a ). Among all unique sequences, 60,732 (60.7%) were found in only one species ( Fig. 8b ). We also observed that conserved, thus abundant, families have a higher number of sequence variants than low abundance families ( Supplementary Data 3 ). This suggested that sequence diversity for a particular family is correlated to its abundance. To test this correlation, we calculated the number of raw reads and the number of distinct sequences for all families in each species. This analysis showed that the number of distinct sequences per family increases as the number of raw reads for all sequences of that family increases, with all species showing an almost identical behaviour ( Fig. 9 ). This is consistent with some of the sequence variants resulting from technical artefacts such as sequencing errors. However, it is also highly likely that some of the sequence variants are new miRNAs. 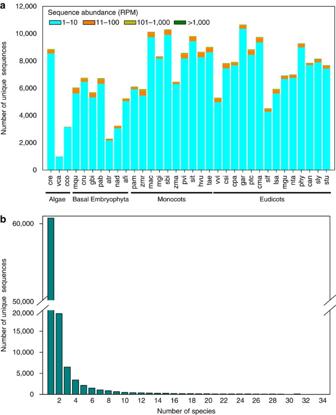Figure 8: The majority of miRNA sequences are of low abundance and present in one species. (a) The majority of miRNA sequences are of low abundance. Stacked bars represent the number of unique miRNA sequences in each species. Each colour represents an abundance category in RPM. (b) The majority of miRNA sequences are present in one species. Bars represent the number of unique sequences present in the corresponding number of species. Figure 8: The majority of miRNA sequences are of low abundance and present in one species. ( a ) The majority of miRNA sequences are of low abundance. Stacked bars represent the number of unique miRNA sequences in each species. Each colour represents an abundance category in RPM. ( b ) The majority of miRNA sequences are present in one species. Bars represent the number of unique sequences present in the corresponding number of species. 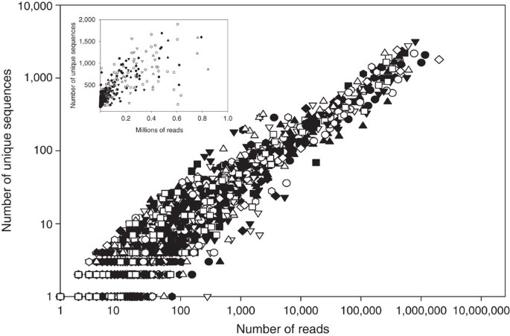Figure 9: Family abundance and sequence variability are correlated. Each data point in the scatter graph represents a miRNA family and each symbol represents a species. Reads are expressed as the sum of raw, non-normalized total reads in all sequencing libraries for a particular family in a particular species. The inset graph uses the same data with a linear scale to show that the correlation is nonlinear, and was truncated at 1 million reads for clarity. Linear regressionR2values for the log-transformed data range from 0.67 to 0.93 with a median of 0.88. In a randomized data set,R2values range from 0.01 to 0.31 with a median of 0.18. Full size image Figure 9: Family abundance and sequence variability are correlated. Each data point in the scatter graph represents a miRNA family and each symbol represents a species. Reads are expressed as the sum of raw, non-normalized total reads in all sequencing libraries for a particular family in a particular species. The inset graph uses the same data with a linear scale to show that the correlation is nonlinear, and was truncated at 1 million reads for clarity. Linear regression R 2 values for the log-transformed data range from 0.67 to 0.93 with a median of 0.88. In a randomized data set, R 2 values range from 0.01 to 0.31 with a median of 0.18. Full size image Identifying putative new miRNA sequences To identify new miRNAs, we performed a relative abundance analysis of all sequences of a particular family. We observed that some sequences were preferentially found in a single species, or in species from a same phylogenetic group. This was clearly illustrated for the miR168-5p family. When the abundance for all miR168-5p sequences is represented in a heatmap and sequences are clustered by abundance, we observe that some sequences are present in distinct phylogenetic groups, three of them immediately apparent, and corresponding to Liliopsida, Solanaceae and non-Liliopsida-non-Solanaceae species ( Fig. 10a ). Then, when the relative abundance of all miR168-5p sequences in each species is plotted, we clearly observe that three sequences are the most abundant in those same Liliopsida, Solanaceae and non-Liliopsida-non-Solanaceae groups, respectively ( Fig. 10b ). The Solanaceae sequence was only recently described in Nicotiana tabacum [31] and could not be found in versions of miRBase prior to 19. This strongly suggests that sequence abundance comparison can be used as a tool to identify putative new miRNA sequences. Indeed, a closer examination of Fig. 10b reveals that the miR168-5p sequences 5′-UCGACUGGUGCAGAUCGGGAA-3′ (present in C. rumphii and G. biloba ), 5′-UCGAUUGGUGCAGAUCGGGAA-3′ ( C. rumphii , G. biloba and P. abies ), 5′-UUGCUUGGUGCAGGUCGGGAA-3′ ( Z. marina ) and 5′-UCGCUUGGUACAGGUCGGGAA-3′ ( Lactuca sativa ) have relative high abundances, and cannot be found in the version 19 release of miRBase. Other examples of putative new miRNA sequences are presented in Supplementary Fig. 8 . 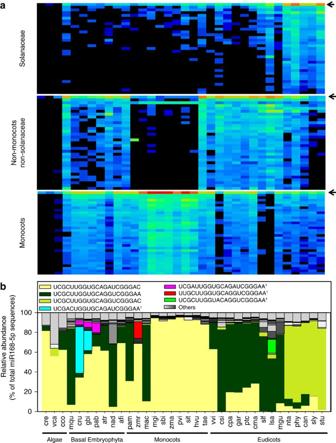Figure 10: Phylogenetic correlations for miR168 sequences. (a) Heatmap for the most abundant sequences of the miR168-5p family. Each row represents a miR168-5p sequence and each column a plant species. Colours correspond to a base 10 logarithm transformation of sequence abundance in RPM, from black (absent) to red (high abundance). Arrows indicate the most abundant sequence in each group. (b) Three distinct miR168-5p sequences represent the majority of miR168-5p sequences. Colour bars represent the relative abundance of miR168-5p sequences. 1, sequences not present in version 19 of miRBase. Figure 10: Phylogenetic correlations for miR168 sequences. ( a ) Heatmap for the most abundant sequences of the miR168-5p family. Each row represents a miR168-5p sequence and each column a plant species. Colours correspond to a base 10 logarithm transformation of sequence abundance in RPM, from black (absent) to red (high abundance). Arrows indicate the most abundant sequence in each group. ( b ) Three distinct miR168-5p sequences represent the majority of miR168-5p sequences. Colour bars represent the relative abundance of miR168-5p sequences. 1, sequences not present in version 19 of miRBase. Full size image Clear examples of new putative miRNA sequences can also be found in species where one or two sequences represent an important proportion of all miRNAs in that species. Figure 7a shows that, in several Tracheophyta species, conserved miRNA families represent a slightly lower proportion of all expressed miRNAs. This is due to the presence of one or two sequences that have very high relative abundances: the miR1083-5p sequences 5′-UAGCCUGGAACGAAGCACGC-3′ (88,409 RPM; 46% of all miRNAs in the species) and 5′-UAGCCUGGAACGAAGCACGGA-3′ (37,446 RPM; 16%) from C. rumphii ; the miR1083-5p sequences 5′-UAGCCUGGAACGAAGCACGU-3′ (35,337 RPM; 22%) and 5′-UAGCCUGGAACGAAGCACGUA-3′ (28,551 RPM; 18%) from G. biloba ; the miR950-5p sequence 5′-UCACGUCAGGGCCACGAUGGUU-3′ (116,302 RPM; 42%) from P. abies ; the miR396-5p sequence 5′-UUCCACGGCUUUCUUGAACUA-3′ (91,736 RPM; 12%) from Z. marina ; the miR5564-5p sequence 5′-UGGGAAGCAAUUCGUCGAACA-3′ (49,408 RPM; 26%) from Sorghum bicolor ; the miR3954_S1 sequence 5′-UUGGACAGAGAAAUCACGGUCA-3′ (31,392 RPM; 16%) and miR156-5p sequence 5′-UUGACGGAAGAUAGAGAGCAC-3′ (20,597 RPM; 10%) from Citrus sinensis ; the miR3954-5p sequence 5′-UUGGACAGAGUAAUCACGGUCG-3′ (38,171 RPM; 30%) from Gossypium arboreum ; and the miR7122-5p sequence 5′-UUAAACAGAGAAAUCGCGGUUG-3′ (9,285 RPM; 7%) from L. sativa ( Supplementary Data 3 ). All these sequences are not present in the version 19 release of miRBase, and their very high abundance in their corresponding species strongly suggests they are true miRNA sequences. For example, the miR156-5p sequence from C. sinensis , 5′-UUGACGGAAGAUAGAGAGCAC-3′, differs in one nucleotide at position 6 from the most abundant miR156-5p sequence 5′-UUGACAGAAGAUAGAGAGCAC-3′ in other species. The fact that it is the second most abundant miRNA sequence in C. sinensis , while it is either absent, or present at low to very low abundances in all other species that we analysed ( Supplementary Data 3 ) strongly suggests that this C. sequence is not a technical artefact derived from the 5′-UUGACAGAAGAUAGAGAGCAC-3′ sequence, but is rather a previously undescribed, bona fide miR156-5p sequence. miRNAs are a class of sRNAs that were first described in animals in 1993 (ref. 32 ) and in plants in 2002 (ref. 33 ). Since then, knowledge of miRNA biogenesis, degradation and biological roles has vastly increased [2] , [34] , [35] . With the advent of next-generation sequencing, an impressive amount of sRNA sequencing data has become publicly available from an ever increasing number of species. While these data have allowed for the identification of new miRNA loci variants from the canonical miRNA sequences that have been termed isomiRs, and non-overlapping miRNAs from the same precursors [36] , [37] , [38] , a comparative analysis of miRNA sequence variation across plant species was still lacking. In this study, we have identified, using miRBase version 19 as a reference, many miRNA sequences present in 99 sequencing libraries from 34 plant species, which allowed us to obtain an overview of miRNA sequences expression and conservation across the plant kingdom. A rather striking result from our data was that a correlation exists between miRNA abundance and conservation in plants ( Fig. 7a,b ). This implies that non-conserved sequences represent a small percentage of all miRNAs, and is consistent with the observation that the majority of miRNA sequences are of low abundance, with 10 or less RPM ( Fig. 8a ). In addition, the low overlap between our identified miRNA sequences and the sequences present in miRBase version 19 suggests that most miRNA sequences are species specific, which is in line with our observation that the majority of miRNA sequences are present in a single species ( Fig. 8b ), and consistent both with previous reports [3] , [5] , [39] , and with the observation that even the closely related species A. thaliana and A. lyrata have each specific miRNAs [6] . In plants, isomiR have been described, for example, in A. thaliana [40] and Prunus persica [41] . However, since the Illumina technology is error prone, isomiR descriptions usually only include sequences that perfectly align to the corresponding reference genome, and thus exclude all substitution variants. Yet 90% of our identified miRNA sequences are substitution variants, and Fig. 9 shows that the number of sequence variants for a particular family is correlated to the number of reads for that same family. It would thus appear that abundance leads to sequence diversity. A simple explanation for this observation would be that the number of sequence variants increases as sequencing events of a particular miRNA sequence occur, that is, a technical artefact. While one would expect the probability of such errors to be sequence dependent, it is possible that miRNA sequences are not significantly biased in nucleotide composition, resulting in a homogenous error rate for all miRNA families, as observed in Fig. 9 . This homogenous correlation in all species and families would therefore suggest that most, if not all, sequence variants are technical artefacts. To differentiate technical artefacts from true miRNA sequence variants, a comparison of the identified miRNA sequences with genome or transcriptome data would be necessary. Genomic data are available for 16 of the species analysed. While the number of identified miRNA sequences that can be found in the genome of the corresponding species is relatively low, they actually represent the majority of reads ( Supplementary Table 1 ). Still, genomic or transcriptomic data are not yet annotated, completed or available for many species that we sampled. In this context, sequence abundance comparison is a powerful alternative for miRNA sequence analysis. In particular, it strongly suggests that previously undescribed, and abundant sequences from a particular species, or a closely related group of species are putative novel miRNA sequences. Sequence abundance comparison also raises interesting questions about miRNA conservation across species. Two examples that illustrate this are the most abundant miR164-5p sequence from basal Embryophyta, and the miR168-5p sequence from Solanaceae species. 5′-UGGAGAAGCAGGGCACGUGCG-3′ is the most abundant miR164-5p sequence in C. rumphii , G. biloba , P. abies , and is also relatively abundant in Nuphar advena and Persea americana . In all other species, it is either absent or has an abundance of less than 5 RPM. Yet this sequence is identical to the miR164c sequence from A. thaliana , thus not exclusive to more basal plant species. The second example concerns the miR168-5p sequence from Solanaceae species. This sequence has an abundance ranging from 982 to 6,821 RPM in Solanaceae species. Interestingly, it can also be found in all 31 Tracheophyta species at low levels, but for some of them at levels that are not insignificant: 26 RPM in M. quadrifolia , 12 RPM in S. bicolor , 10 RPM in Panicum virgatum , 37 RPM in Hordeum vulgare , 60 RPM in Musa acuminata , 77 RPM in C. sinensis , 18 RPM in Carica papaya , 23 RPM in Cucurbita maxima , 92 RPM in S. latifolia , 347 RPM in L. sativa and 15 RPM in M. guttatus . The presence of this sequence across the plant kingdom would suggest that it originated early during Tracheophyta evolution, and is preferentially expressed in Solanaceae species. We propose two possible origins for such sequences that belong to conserved families, and exhibit this high-abundance/low-abundance/absence behaviour across species. One possibility is that such sequences represent loci that are preferentially expressed in some species, but are downregulated, or completely lost, in other species. The above-mentioned miR164-5p and miR168-5p sequences are examples that fit this scenario. A second possibility is suggested by the results from analyses by Breakfield et al. [40] of cell type-specific miRNAs in A. thaliana roots. Their results have shown that non-canonical sequences, that is, miRNAs that do not correspond to the sequence found in the TAIR or miRBase databases can be the most abundant miRNAs for a particular family in a particular A. thaliana root cell type. In a global tissue analysis (whole root, whole leaf and so on), such as those that we have developed, we expect a dilution of these cell type-specific miRNAs to occur, and these sequences would then be detected at low abundances. Regardless of their origin, the presence of low-abundance sequences raises the question of their biological relevance. miRNA depletion experiments have been carried out for conserved or highly conserved families, and have shown that such families play relevant roles during plant development [42] , [43] . However, depletion of low-abundance, non-conserved miRNA families has not yet been performed. It is therefore unclear whether the biological role of a miRNA is a function of its abundance, or whether a difference exists between the type of target genes regulated by high- versus low-abundance miRNAs from the same family. Since conserved families represent the majority of total miRNA abundances, sequences present in one to a few species will most probably be present in low abundance. This is for example the case for the miR1916, miR1917, miR1918 and miR1919 families, first described in Solanum lycopersicum [39] and present in other Solanaceae species with a low overall abundance ( Supplementary Data 3 ). While lineage-specific miRNAs would appear to lack target mRNAs [7] , [12] , target genes for the S. lycopersicum miRNA families were validated by 5′-rapid amplification of cDNA Ends and their expression is higher in mature fruits than younger fruits [39] , which points to these miRNAs as having a role in a developmental process, namely, fruit ripening. This would suggest that other low-abundance sequences, from either conserved or non-conserved families, could also have relevant biological functions. Finally, our results, and those of others [40] , raise the question of the definition of ‘canonical’ sequence and, by extension, the definition of ‘isomiR’. These data show that the most abundant sequences can vary across species or across cell types in the same organ of a particular species, and can be absent from databases such as miRBase. It would therefore appear that ‘canonical’ sequence will have to be defined on a case by case basis as the most abundant sequence for a particular family in a particular species/organ/cell type/developmental stage. In summary, this work represents a massive atlas of sRNA and miRNA expression across a diverse panel of 34 plant species, including non-model plants. By greatly enhancing the depth and breadth of plant sRNA sequencing and analysis available to date, this study provides new insights and a resource that will be beneficial well into the future. Plant material Plant material was obtained from 99 different tissue samples from 34 species as indicated in Supplementary Data 1 . Total RNA was isolated from each of the 99 samples using the Plant RNA Purification Reagent (Invitrogen), TRiReagent/TRIzol (Molecular Research Center/Invitrogen) or guanidinium-free RNA isolation protocols. The detailed procedures can be found in ref. 44 . In most cases, RNA was submitted to Illumina (Hayward, CA, http://www.illumina.com ) for sRNA library construction, using approaches described in ref. 45 with minor modifications, and sequenced. For C. corallina sample 1 and Petunia hybrida sample 1, sRNA libraries were constructed in house and sequenced on an Illumina Genome Analyzer II at the Delaware Biotechnology Institute. Data availability Sequence data have been deposited in NCBI’s Gene Expression Omnibus and are accessible through GEO Series accession number GSE28755 ( http://www.ncbi.nlm.nih.gov/geo/query/acc.cgi?acc=GSE28755 ) and also can be accessed from the Comparative Sequencing of Plant Small RNAs database [46] at the website http://smallrna.udel.edu/ . The analysed data consisted of 99 trimmed sRNA libraries. MiRBase mature miRNA sequences, version 19, were obtained from the miRBase [20] website ( http://www.mirbase.org/ ). Identification of miRNA sequences To compare our sRNA sequences with miRBase mature miRNA sequences, we collapsed the miRBase version 19 entries to obtain a list of unique sequences. As the information provided by miRBase nomenclature was not always sufficient to distinguish sequences belonging to the same miRNA family but deriving from different regions of a precursor, we used a custom pipeline to separate sequences from each family into distinct groups by sequence similarity, and assigned to each of these groups a random suffix in the form of _S1, _S2 and so on. For miRNAs analysed and discussed in greater detail in the text, the suffixes were replaced with 3 p and 5 p designations, determined from manual analysis. Then, to identify miRNA sequences present in our PSRNAdb sequencing libraries, we aligned the library sequences to our modified miRBase reference set using the program seqmap, version 1.0.13 (ref. 47 ). Seqmap is an end-to-end mode aligner and, therefore, query sequences with extra bases, or shifted, relative to the mature miRBase sequences, will be missed. To avoid this, we used a different version of our miRBase reference set where each individual sequence was modified by the addition of two nucleotides at both the 5′- and 3′-ends, with all possible combinations of dinucleotides added. This transforms each collapsed miRBase sequence into 256 (4 4 ) different modified sequences. The resulting modified miRBase fasta file was used as reference for seqmap. The command line used was seqmap 3 input_file.fasta miRBase.fasta output_file.txt/forward-strand/output-all-matches. The parameter ‘3’ allows up to three mismatches. Individual seqmap reports were parsed using custom Perl scripts to retrieve, for each sRNA, the corresponding best matching miRBase miRNA. When a sRNA sequence matched two, or more, miRBase sequences from different families, the best match was determined as the alignment that contained fewer mismatches, and was centred on the original miRBase sequence (that is, was not shifted). If, after these consecutive criteria, a sequence equally matched two or more miRBase sequences from different families, it was considered an ambiguous sequence and was discarded, except sequences matching either the miR156_S2 (5p) and miR157_S2 (5p) families, or the miR165_S1 (3p) and miR166_S1 (3p) families, which were particularly abundant. All miR156_S2 (5p) and miR157_S2 (5p) sequences were named miR156_S2 (5p), and all miR165_S1 (3p) and miR166_S1 (3p) sequences were named miR166_S1 (3p). Initial seqmap runs indicated that the PSRNAdb sequencing libraries contain sRNA sequences that match animal or virus miRNA sequences. The existence of miRNAs conserved between animals (or viruses) and plants was puzzling. However, we noticed that animal (or virus) miRNA sequences in PSRNAdb libraries were almost always present in very low read numbers, usually 10 reads or lower. It was also apparent that miRNA sequences well represented in the animal kingdom were present in most of the PSRNAdb plant species, while sequences only present in a few animal species were sparsely present in PSRNAdb plant species. These observations strongly suggested contamination of the plant samples, either during collection of the biological material or cross-contamination during sequencing. Thus, our data provide no support for conserved miRNA sequences between animals/viruses and plants, consistent with other indications in the literature [2] , [4] , [48] . To avoid the recovery of animal or virus sequences, the modified miRBase file was filtered and only entries from Viridiplantae species were kept. This Viridiplantae-specific miRBase file was then used as reference for seqmap runs. After parsing of the seqmap output files, using a sequence length cutoff of 18–26 nucleotides, we obtained the list of identified miRNAs for all 34 PSRNAdb species. Ambiguous sequences represented a mere 17,829 reads, from a total of over 36 million miRNA reads, and thus could be safely discarded. As the vast majority of our identified miRNA sequences were in the 20–24 nucleotide-long range ( Supplementary Fig. 9 ), the fasta file was filtered to keep only sequences in this size range. Finally, only sequences with at least two reads across all 99 libraries were kept. The resulting fasta file ( Supplementary Data 2 ) was used for all subsequent analyses. Each sequence name in this file is in the form [species]-[miRNA family]_[sample id]-[id]-[reads]_[mismatches], where [species] and [sample_id] correspond to the three-letter and one-digit codes of the corresponding PSRNAdb library file name ( Supplementary Data 1 ), [id] is an arbitrary number for each sequence, [reads] is the number of reads for that sequence and [mismatches] is the number of mismatches relative to its miRBase match. For example, a sequence with the name afi-miR156_1-559870-4_1 corresponds to a sequence from the afi1 library, matching a miR156 miRBase miRNA sequence, with the arbitrary id number 559870, four reads in that library and one mismatch relative to its matching miRBase sequence. For two species, PSRNAdb three-letter codes conflicted with miRBase codes: ptr, Populus trichocarpa in PSRNAdb, is Pan troglodytes in miRBase and sla, S. latifolia in PSRNAdb, is Saguinus labiatus in miRBase. We therefore changed the three-letter code to ptc for P. trichocarpa and to slf for S. latifolia . Three-letter codes for all PSRNAdb species are indicated in Fig. 1 and Supplementary Data 1 . Abundance normalization Trimmed sRNA sequencing libraries were aligned versus a database of ribosomal RNA, transference RNA, small nuclear RNA and snoRNA, and versus a modified (see above) miRBase reference file containing only animal and virus sequences. The total number of reads for sequences matching either r/t/sn/snoRNAs, or animal and virus miRNAs in each sequencing library was calculated. This total was then subtracted from the total library size and the resulting number was used for abundance normalization ( Supplementary Table 2 ). Abundances are expressed throughout this work in RPM unless otherwise indicated. Alignment to genomic sequences Genomic data for 16 species ( C. reinhardtii [49] , V. carteri [50] , M. acuminata [51] , S. bicolor [52] , Zea mays [53] , P. virgatum ( http://www.phytozome.net/dataUsagePolicy.php?org=Org_Pvirgatum_v1.1 ), S. italica [54] , H. vulgare [55] , T. aestivum ( http://www.wheatgenome.org/ ), V. vinifera [56] , C. sinensis , C. papaya [57] , P. trichocarpa [58] , M. guttatus ( http://www.phytozome.net/dataUsagePolicy.php?org=Org_Mguttatus_v2.0 ), S. lycopersicum [59] and S. tuberosum [60] ) was downloaded from Phytozome [61] or EnsemblPlants [62] . Identified miRNA sequences from the corresponding species were aligned using bowtie [63] with the parameters -a and -v 0, and output files were parsed with a custom Perl script to retrieve the names and number of reads of the sequences that perfectly aligned to the genome. Accession codes: The sequence data have been deposited in the NCBI Gene Expression Omnibus under accession code GSE28755 . How to cite this article: Chávez Montes, R. A. et al. Sample sequencing of vascular plants demonstrates widespread conservation and divergence of microRNAs. Nat. Commun. 5:3722 doi: 10.1038/ncomms4722 (2014).